A green lead hydrometallurgical process based on a hydrogen-lead oxide fuel cell The automobile industry consumed 9 million metric tons of lead in 2012 for lead-acid batteries. Recycling lead from spent lead-acid batteries is not only related to the sustainable development of the lead industry, but also to the reduction of lead pollution in the environment. The existing lead pyrometallurgical processes have two main issues, toxic lead emission into the environment and high energy consumption; the developing hydrometallurgical processes have the disadvantages of high electricity consumption, use of toxic chemicals and severe corrosion of metallic components. Here we demonstrate a new green hydrometallurgical process to recover lead based on a hydrogen-lead oxide fuel cell. High-purity lead, along with electricity, is produced with only water as the by-product. It has a >99.5% lead yield, which is higher than that of the existing pyrometallurgical processes (95–97%). This greatly reduces lead pollution to the environment. With the rapid developments in the automobile industry, the production of lead (Pb)-acid batteries as the automotive ignition power source has experienced enormous growth during the past few decades [1] . In 2012, 9 million metric tons of refined Pb, which is about 85% of annual Pb production, was consumed globally for manufacturing Pb-acid batteries for vehicles ( http://www.ilzsg.org/static/statistics.aspx?from=1 ). Moreover, due to their low cost, Pb-acid batteries are also a strong contender for grid storage of electricity produced by renewable energies such as solar and wind. An annual growth rate of >6% is anticipated for the production of refined Pb. Although there is no Pb pollution from using Pb-acid batteries, their widespread use has caused a severe environmental problem due to toxic Pb emission and high energy consumption of the existing Pb pyrometallurgical processes for preparing metallic Pb [2] . The raw materials (lead compounds) of the existing Pb pyrometallurgical processes are mainly obtained by extraction from natural lead oxide ores and pre-roasting oxidation of galena (lead sulphide (PbS)→lead oxide (PbO)). As Pb-acid batteries have been used worldwide in vehicles for decades, the raw materials are now mainly attained by recovering from waste Pb-acid batteries via the desulfurization process of lead sulphate (PbSO 4 ) [3] , [4] and the redox reaction of Pb and lead dioxide (PbO 2 ) [5] , [6] . The pyrometallurgical processes employ coke or carbon monoxide to reduce lead compounds at high temperature (about 1,000 °C) to gain the crude Pb with the release of CO 2 gas [7] . Pb vapour/dust is also produced owing to its low melting point and escapes along with the exhaust gases into the atmosphere, known as Pb pollution [7] , [8] , [9] . High-purity Pb (99.99%) is then obtained by refining the crude Pb using electrolytic refining or fire refining [8] . The whole process has a yield of 95–97% (refs 7 , 9 , 10 ). Hydrometallurgical processes were proposed to eradicate the Pb pollution problem and obtain high-purity Pb (99.99%) without the refining step [8] , [11] , [12] , [13] , [14] , [15] , [16] , [17] , [18] , [19] , [20] . These processes do not emit Pb vapour/dust to the environment due to their low operating temperature and lack of vapour production [8] , [11] ; however, there are still many disadvantages, such as high electricity consumption, use of highly toxic hexafluorosilicic acid electrolyte and severe corrosion of metallic components [12] , [13] , [14] , [15] , [16] , [17] , [18] , [19] , [20] , [21] . As a result, these processes have not yet been adopted by the industry. It is an urgent requirement to develop a new green lead recovery process with lower energy consumption and without the use of toxic chemicals. Herein we report a new green hydrometallurgical process for producing high-purity metallic Pb based on a specially designed H 2 –PbO fuel cell. The PbO serves as the Pb source and is pre-refined in a hot sodium hydroxide (NaOH) aqueous solution. This and the hydrogen gas undergo electro-reduction at the cathode and electro-oxidation at the anode in the fuel cell, respectively. The new process is energy-efficient and toxic-free (except for PbO and Pb), and it produces only Pb, water and electricity. It also does not involve Pb emission due to the low operating temperature of 60–100 °C. The NaOH concentration, temperature, PbO concentration and current density have been optimized to synthesize a dense, high-purity Pb (99.9992%), qualified for Pb-acid batteries with a high yield of 99.5–99.8%, which is higher than that of existing pyrometallurgical processes (95–97%), and greatly reduces lead pollution to the environment. 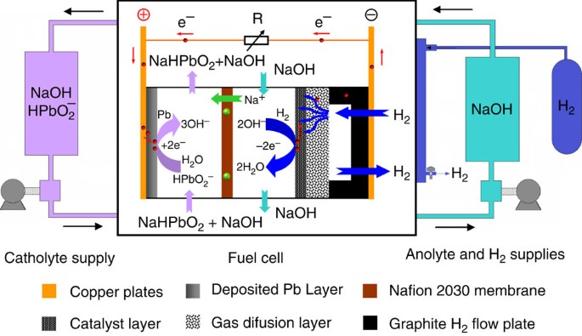Figure 1: Schematic of the H2–PbO fuel cell. The Nafion 2030 membrane (DuPont) is an ion-selective, reinforced composite membrane designed to transport sodium ions and water while blocking OH−and HPbO2−ions. The diffusion layer is a carbon paper (TGP-H-060, Toray) coated with carbon black (Vulcan 72 R, Cabot). The catalyst is carbon black-supported platinum nanoparticles (40 wt% Pt/C, Johnson Matthey). H 2 –PbO fuel cell Figure 1 illustrates the schematic of the new green hydrometallurgical process using the proposed H 2 –PbO fuel cell. Hydrogen gas is fed into the anode, where it undergoes electro-oxidation with the OH − ions to form water and releases electrons. The electrons pass through the external circuit, carry out electric work, and then arrive at the cathode. The refined PbO dissolved in heated aqueous NaOH forms HPbO 2 − ions, which are then pumped into the cathode, where the HPbO 2 − ions combine with the electrons from the anode and water to produce metallic Pb and OH − ions. The produced OH − ions combine with the Na + ions migrating from the anolyte through the sodium-ion exchange membrane to form NaOH. The involved reactions including the complexation dissolution of PbO in NaOH are given below: Figure 1: Schematic of the H 2 –PbO fuel cell. The Nafion 2030 membrane (DuPont) is an ion-selective, reinforced composite membrane designed to transport sodium ions and water while blocking OH − and HPbO 2 − ions. The diffusion layer is a carbon paper (TGP-H-060, Toray) coated with carbon black (Vulcan 72 R, Cabot). The catalyst is carbon black-supported platinum nanoparticles (40 wt% Pt/C, Johnson Matthey). Full size image Anode: H 2 +2OH − →2H 2 O+2e − (electro-oxidation, E °=−0.828 V) Cathode: PbO(s)+OH − →HPbO 2 − (complexation reaction) HPbO 2 − +2e − +H 2 O→Pb(s)+3OH − (electro-reduction, E °=−0.531 V) The overall reaction of the fuel cell is H 2 +PbO(s)→H 2 O+Pb(s) (E°=−0.531−(−0.828)=0.297 V) The positive standard potential of 0.297 V means that the reaction between H 2 and PbO occurs spontaneously to produce Pb, water and electricity. The experimental results show that the open-circuit voltage at room temperature is 0.226 V, which is a little lower than the standard potential due to the non-standard conditions such as temperature, concentration and small polarization losses. The complexation dissolution of PbO in a hot aqueous NaOH solution has a key role in making this process feasible. Although PbO is generally considered a basic metal oxide, it has a high solubility in concentrated aqueous NaOH solutions [22] . As shown in Fig. 2 , the solubility of PbO strongly depends on temperature when the NaOH concentration is above 15%. This characteristic of its solubility makes it possible to obtain a high concentration of high-purity PbO by a recrystallization process, which produces high-purity Pb at a fast reaction rate. 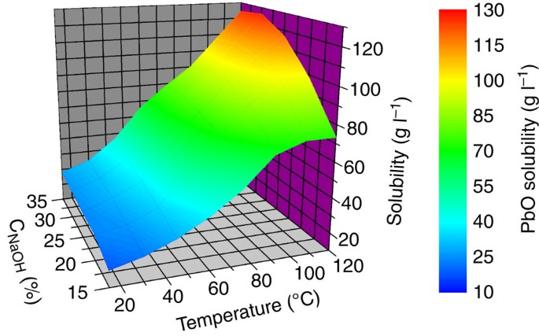Figure 2: Solubility of PbO versus temperature and NaOH concentration. The solubility is determined by a complexometric titration with EDTA. Figure 2: Solubility of PbO versus temperature and NaOH concentration. The solubility is determined by a complexometric titration with EDTA. Full size image PbO recovery and purification The PbO in this study was recovered from the spent lead paste (Zhejiang Huitong Group) from used Pb-acid batteries by a desulfurization process of lead sulphate and a redox reaction of Pb and PbO 2 with a catalyst [6] . The actual recovery efficiency of PbO reaches 99.7%. The recovered PbO was purified by a recrystallization process, which is based on the strong temperature dependence of PbO solubility in a concentrated aqueous NaOH solution. The high purity of the obtained PbO ensures the quality of the electrolyte and the Pb synthesized by a H 2 –PbO fuel cell. 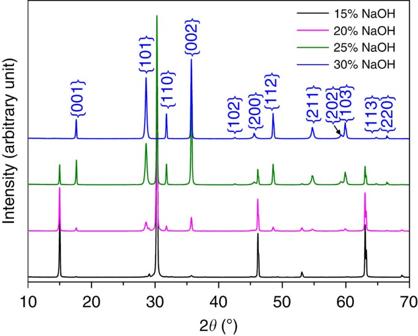Figure 3: XRD patterns of the PbO samples. The purified PbO samples were obtained from different concentrations of NaOH solutions: 15, 20, 25 and 30%. Figure 3 compares the XRD patterns of the PbO samples purified by recrystallization in different concentrations of NaOH. The location of the {001} peak was used to identify the polymorph of the PbO phase, that is, massicot or litharge. It was found that the PbO obtained from a low concentration of NaOH (15%) is massicot (PDF no. 00-005-0570) and from a high concentration (30%) is litharge (PDF no. 00-005-0561). The PbO obtained from NaOH concentrations of 15–30% is a mixture of massicot and litharge. It was also found that the PbO obtained in 30% NaOH has the main peak located at about 35.7°, which means that the crystalline PbO prefers to grow along with <002> direction. Figure 3: XRD patterns of the PbO samples. The purified PbO samples were obtained from different concentrations of NaOH solutions: 15, 20, 25 and 30%. Full size image All purified PbO samples show irregular shapes with sizes in the range of 10–15 μm ( Supplementary Fig. S1 ). Compared with the desulfurized PbO from the spent lead-acid batteries, the inductively coupled plasma (ICP) analysis shows that the purified PbO samples have much lower impurities of other metals ( Table 1 ). These high-purity PbO samples are suitable for the synthesis of high-quality Pb. Table 1 ICP analysis results of the PbO samples. Full size table Synthesis of metallic Pb The first trial to obtain Pb was carried out with an anolyte of 20% NaOH and a catholyte of 20% NaOH+0.1 mol l −1 PbO at a current density of 5 mA cm −2 at room temperature. The XRD pattern in Fig. 4a confirms that the obtained grey material on the copper cathode is metallic Pb with some PbO impurities. The sample is made of loose particles as shown in the field emission-scanning electron microscopy (FE-SEM) image in Fig. 4b . Compared with bulk dense Pb, this particulate Pb has a larger surface area and is thus easier to oxidize in air in storage and in the melting process to make lead ingots. This is why some PbO co-exists as shown by the XRD pattern in Fig. 4a . The product is also porous with a large volume, which is not desirable for transport and storage. 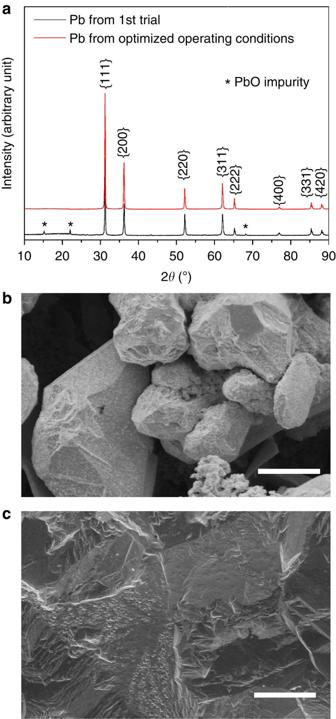Figure 4: Pb samples produced in the H2–PbO fuel cell. (a) X-ray diffraction patterns of the Pb samples produced initially and under optimized conditions later. (b) FE-SEM image of the Pb sample produced initially. (c) FE-SEM image of the Pb produced under optimized conditions. Scale bar, 100 μm. Figure 4: Pb samples produced in the H 2 –PbO fuel cell. ( a ) X-ray diffraction patterns of the Pb samples produced initially and under optimized conditions later. ( b ) FE-SEM image of the Pb sample produced initially. ( c ) FE-SEM image of the Pb produced under optimized conditions. Scale bar, 100 μm. Full size image To obtain high-purity Pb with a dense structure, fast reaction rate and high yield, three factors, the NaOH concentration (same at the anode and cathode before operation, 15–35%), temperature (30–105 °C) and PbO concentration (0.05–0.4 mol l −1 ), were systematically investigated. The details are presented in Supplementary Notes 1,2,3 , respectively. A brief description is given as follows. A low NaOH concentration is favourable to the formation of a dense structure ( Supplementary Fig. S2 ) and the kinetics of the electro-reduction reaction of Pb 2+ ( Supplementary Fig. S3 ). As for the temperature effects, an intermediate temperature is helpful to form a dense structure ( Supplementary Fig. S4 ). A high temperature increases the kinetics of the electro-reduction reaction of Pb 2+ ( Supplementary Fig. S5 ) and the hydrogen electro-oxidation reaction ( Supplementary Fig. S6 ). A comparison between the kinetics of both reactions ( Supplementary Fig. S7 ) reveals that the H 2 –PbO fuel cell performance is limited by the Pb 2+ electro-reduction. Similar to the temperature effect, an intermediate PbO concentration helps form a dense structure ( Supplementary Fig. S8 ) and a high PbO concentration promotes the kinetics of the electro-reduction reaction of Pb 2+ ( Supplementary Fig. S9 ). All three factors do not significantly affect the current efficiencies of the Pb electro-deposition, as shown in Supplementary Tables S1,S2,S3 , respectively. Considering the morphology of the produced Pb (dense structure), the kinetics of the Pb electro-deposition reaction (low overpotential and fast reaction) and the current efficiency, the optimized NaOH concentration, temperature and PbO concentration were determined to be 20%, 85 °C and 0.3 mol l −1 , respectively. The Pb prepared under the optimized conditions has a dense structure (FE-SEM image in Fig. 4c ) and thus has no significant oxidation, as confirmed by the XRD pattern in Fig. 4a . The ICP analysis in Table 2 indicates that the purity of the electro-deposited Pb is 99.9992%, which is much higher than the 1# standard Pb (GB/T 468-2005, Chinese standard, 99.994%) and PB990R grade Pb (EN 12659-1999, European standard, 99.99%). This ultra-high-purity Pb is a superior material for the manufacture of high-quality Pb-acid batteries with a longer cycle life. In addition, all of the current efficiencies are greater than 99.5%, indicating a very high selectivity of the Pb reduction reaction at the cathode. Table 2 Comparison of Pb compositions. 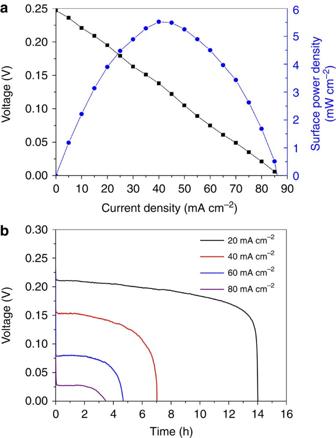Figure 5: Characterizations of the new lead hydrometallurgical process. (a) Polarization curve and specific power curve of the H2–PbO fuel cell. (b) Voltage versus time curves at different current densities of the H2–PbO fuel cell. Full size table Figure 5a shows the polarization curve and surface power curve of the H 2 –PbO fuel cell operated under the optimized conditions. The Pb samples prepared at 20, 40, 60 and 80 mA cm −2 have dense structures as shown by the FE-SEM images ( Supplementary Fig. S10 ), suggesting that the current density does not affect the surface morphology of the Pb samples. Additionally, the current density also does not affect the current efficiency ( Supplementary Table S4 ). Therefore, the fuel cell can operate at 40 mA cm −2 to achieve a maximum electric surface power density of 5.5 mW cm −2 at 80 mA cm −2 and a high production rate of Pb. As shown in Fig. 5b , the reduction of PbO can be accomplished in 14.02, 7.02, 4.69 and 3.45 h at 20, 40, 60 and 80 mA cm −2 , respectively. According to Faraday’s law, the reaction conversions of PbO to Pb were 99.6%, 99.8%, 99.7% and 99.3%. The catholyte thus had a very small amount of unreacted PbO residue. This residual PbO can be further reduced by an ion exchange process or electrolysis until it does not affect the recyclability of the reacted catholyte for preparing the anolyte. Figure 5: Characterizations of the new lead hydrometallurgical process. ( a ) Polarization curve and specific power curve of the H 2 –PbO fuel cell. ( b ) Voltage versus time curves at different current densities of the H 2 –PbO fuel cell. Full size image This new green Pb hydrometallurgical process employing an H 2 –PbO fuel cell eliminates Pb pollution and significantly reduces energy consumption, which are the two major issues for the existing Pb pyrometallurgical processes and other developing pyrometallurgical and hydrometallurgical processes. A detailed comparison is given in Table 3 . Unlike the pyrometallurgical processes, this new process has no Pb vapour or slag released to the environment, leading to an annual reduction of 12,000–20,000 metric tons of Pb (vapor/dust and slag) emission to the environment for a plant with an annual output of 400,000 metric tons of Pb. Furthermore, compared with other hydrometallurgical processes, this new process does not employ any toxic chemicals, such as hydrofluoric acid. Regarding the energy consumption, this new process needs about 1/2 or 1/3 of the energy used for the existing pyrometallurgical or other hydrometallurgical processes, respectively. This new process, as a fuel cell, also produces electricity (5.3–45.5 W h per kg of Pb) depending on the current density, and can also be applied for preparation of other metals such as copper, silver, antimony and nickel. To accomplish this, two main conditions need to be satisfied. First, the raw materials should dissolve in a basic solution. Second, the reduction potential of the metal ions should be higher than that of the hydrogen ion. Table 3 Comparison of three Pb metallurgical processes. Full size table General procedure for recovery of PbO from the spent lead paste The spent lead paste from used Pb-acid batteries was supplied by Zhejiang Huitong Group, China. Its main ingredients are 12.6% Pb, 15.3% PbO, 26.8% PbO 2 and 44.2% PbSO 4 , and the remainder (1.1%) is H 2 O and H 2 SO 4 . The recovery of PbO from the spent lead paste employs four processes [6] : desulfurization , redox, synchronizing dissolution and crystallization. The involved chemical reactions and detailed descriptions are given below. Desulfurization process PbSO 4 (s)+2NaOH(aq)=PbO(s)+H 2 O+Na 2 SO 4 (s) (30 °C). The spent lead paste (100 g) was added to 10% NaOH (120 ml) for the desulfurization process to convert PbSO 4 to PbO. The reaction temperature was controlled at 30 °C and the paste was stirred at 150 r.p.m. for 10 min. Redox process Pb(s)+PbO 2 (s)+2NaOH(aq)=2NaHPbO 2 (aq) (115 °C). The obtained sample A (a mixture of Pb, PbO and PbO 2 ) from the desulfurization process was filtered with a Buchner funnel and washed with deionized water. Sample A was carefully transferred to the reactor containing 30% NaOH saturated with 30 g l −1 PbO at room temperature. A calculated amount of Pb powder (10.6 g, 120 mesh) was supplied as the reductant and Na 3 SbO 3 (0.15 g) was added as the catalyst for the redox reaction of Pb and PbO 2 . The reaction was controlled at 115 °C and the reaction paste was stirred at 300 r.p.m. for 3 h. Synchronizing dissolution process PbO(s)+NaOH(aq)=NaHPbO 2 (aq) (115 °C). During the redox process, the PbO of sample A was also synchronization dissolved in the NaOH solution at 115 °C. Crystallization process NaHPbO 2 (aq)=NaOH(aq)+PbO(s) (25 °C). The previously obtained NaHPbO 2 /NaOH solution was immediately filtered and slowly cooled to room temperature with continuous stirring. During the cooling process, kermesinus PbO slowly precipitates from the solution. It was filtered by a G-2 sintered glass filter, washed with deionized water and dried at 60 °C. The final recovered PbO weighed 97.2 g, and thus the PbO recovery efficiency was 99.7%. Determination of PbO solubility The recovered PbO was purified by a recrystallization process. The solubility of the purified PbO in NaOH aqueous solutions was determined by a complexometric titration with EDTA, described as follows. An excess of PbO was added to a NaOH solution, which was then stirred and heated to the temperature, at which the solubility will be determined. The solution was kept stirring at that temperature for 5 min and subsequently stayed still for 10 min. An aliquot of this PbO/NaOH solution (0.10 ml) was quickly transferred to a stirring HNO 3 solution (10 ml, 1 mol l −1 ). After that, an extra amount (1.5 × stoichiometric amount) hexamethylenetetramine was added to neutralize the HNO 3 . The solution was finally titrated by a standard EDTA solution (0.020 mol l −1 ) with xylenol orange as the indicator. H 2 –PbO fuel cell and synthesis of Pb The H 2 –PbO fuel cell consisted of an anode of 2 × 2 cm 2 carbon paper (TGP-H-060, Toray) with a carbon black (Vulcan 72R, Cabot) loading of 0.5 mg cm −2 and a Pt catalyst loading of 1.0 mg cm −2 (40 wt% Pt/C, Johnson Matthey) [23] , a cathode of 2 × 2 cm 2 high-purity copper plate, Nafion 2030 sodium ion-selective membrane (DuPont), anolyte of aqueous NaOH solution (15–35%, 60 ml min −1 ) and catholyte of aqueous NaOH–PbO (15–35% NaOH and 0.05–0.4 mol l −1 PbO, 60 ml min −1 ) solution. The NaOH concentrations at the anode and cathode were kept the same before operation. The H 2 flow rate was kept at about 5 ml min −1 for 30 min to expel the air in the hydrogen channel before operation. The valve at the hydrogen channel outlet was closed during the experiments. The pressure of H 2 in the channel was 0.1 MPa. To reduce the formation of Pb dendrites, DPE-3 (electroplating additive, Wuhan Yangtze Plating Additives Plant) was added as an additive into the catholyte with a concentration of 6 ml l −1 . Two Hg/HgO reference electrodes were used to control the potentials of the anode and cathode. A battery test station (LAND 2001A, Wuhan LAND Electronics) was used to run the fuel cell in constant current mode. The electrochemical measurements of the fuel cell were performed on a CSU-300 electrochemical workstation (Wuhan Corrtest Instrument). Characterization of the synthesized Pb For the characterization of the Pb product, the cathode with produced Pb plate was taken out from the system, washed with deionized water, vacuum dried at 60 °C for 3 h and then stored under argon to avoid oxidation in air. The mass of Pb was obtained by subtracting the Cu cathode from the total mass of the Cu cathode with Pb. The Pb surface morphology was examined by an FE-SEM (Hitachi S4700). The composition of the Pb was measured with an ICP analyzer (Agilent 7700). The XRD patterns of the Pb samples were recorded on a Rigaku D/max2500VB2+/PC diffractometer with Cu Kα radiation ( λ =0.15418, nm, 40 kV, 200 mA). How to cite this article: Pan, J. et al . A green lead hydrometallurgical process based on a hydrogen-lead oxide fuel cell. Nat. Commun. 4:2178 doi: 10.1038/ncomms3178 (2013).